MOBILE pipeline enables identification of context-specific networks and regulatory mechanisms 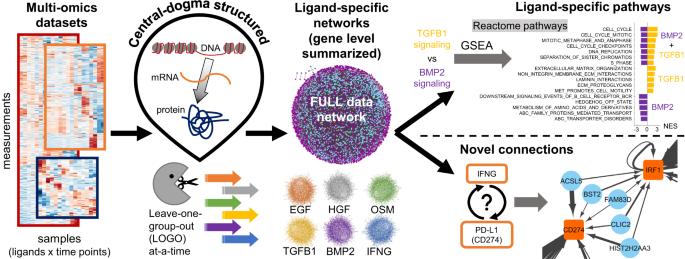Fig. 1: Multi-Omics Binary Integration via Lasso Ensembles (MOBILE) pipeline yields statistically robust, ligand-specific association networks. The MOBILE data integrator combines multi-omics, multi-assay datasets in a data-driven and central-dogmatic way. By leaving each ligand condition out from the input at a-time, the pipeline outputs robust ligand-specific association networks. These gene-level networks are used to infer differentially enriched pathways and to find regulatory sub-networks. Robust identification of context-specific network features that control cellular phenotypes remains a challenge. We here introduce MOBILE (Multi-Omics Binary Integration via Lasso Ensembles) to nominate molecular features associated with cellular phenotypes and pathways. First, we use MOBILE to nominate mechanisms of interferon-γ (IFNγ) regulated PD-L1 expression. Our analyses suggest that IFNγ-controlled PD-L1 expression involves BST2 , CLIC2 , FAM83D , ACSL5 , and HIST2H2AA3 genes, which were supported by prior literature. We also compare networks activated by related family members transforming growth factor-beta 1 (TGFβ1) and bone morphogenetic protein 2 (BMP2) and find that differences in ligand-induced changes in cell size and clustering properties are related to differences in laminin/collagen pathway activity. Finally, we demonstrate the broad applicability and adaptability of MOBILE by analyzing publicly available molecular datasets to investigate breast cancer subtype specific networks. Given the ever-growing availability of multi-omics datasets, we envision that MOBILE will be broadly useful for identification of context-specific molecular features and pathways. The availability of large-scale multi-omics datasets across cell types, tissues, and organisms is rapidly increasing with the development of new technologies [1] , [2] , [3] , [4] , [5] , [6] , [7] . The challenge now is in analyzing them, not individually, but rather together to leverage the fact that signals are encoded across multiple modalities [8] , [9] , [10] , [11] . Examples of individual methods include: principal components analysis [12] , statistical approaches [13] , [14] , [15] , clustering [16] , [17] , [18] , [19] , unsupervised learning [20] , and supervised/machine learning [10] , [21] , [22] , [23] , [24] . Often, such analyses are used to generate networks where genes (or other biomolecules) are nodes, and edges between them denote statistical or functional relationships. Integrating data from multiple modalities can give rise to novel biological insights that cannot be obtained through the analysis of single datasets [25] , [26] , [27] . To date, data integration methods have produced systems-level biological insights, including genetic and protein–protein interactions [28] , [29] , [30] , disease-gene relationships [24] , [31] , drug response predictions [30] , [32] , and context-specific associations [29] , [31] , [33] . A central problem in network biology is the identification of “context-specific” networks. Here we define context-specificity as a biological relationship (i.e., edge in a network) that applies only to a certain cell type, ligand perturbation, extracellular matrix component, or time point. Data integration has the potential to lead to significant advances in our understanding of such context-specific biology by identifying biological signals evident across multiple modalities [8] . For instance, why does insulin, but not insulin-like growth factor I (IGF1), regulate glucose metabolism despite their textbook signaling pathways being essentially identical [34] , [35] , [36] ? Why does IGF1 activate ERK or AKT signaling only in certain cell types [37] , [38] ? Identifying and studying context-specific observations is important because most diseases are tissue-specific [39] , and this knowledge can enable understanding of how different cell types respond to varied perturbations, which is key to targeted therapeutic intervention. Multiple data integration methods have been implemented using bioinformatics tools, including kernels [40] , [41] , correlation analysis [42] , [43] , [44] , [45] , and others [46] . These methods were applied -but not limited- to processing genomic and epigenomic datasets to cluster and classify the input data. Published methods also include network (protein–protein or genomic interaction) inference using omics datasets, including Bayesian approaches [47] , [48] and natural language processing [49] . One group of data integration approaches use prior literature/network knowledge as an essential first step [28] , [29] , [30] , [31] , [32] , [33] , [50] , [51] , [52] , [53] . For example, a prior knowledge-informed network analysis may limit exploration to curated pathways and remove analytes (measured features) with no known interactions, or may impose biological structure into the underlying network models [29] , [30] . These literature-driven approaches assemble available tissue-specific expression data into gene correlation networks [30] , [54] , [55] or overlay the data on global (non-specific) interaction networks [9] , [28] , [56] . For instance, employing a network/graph theory-based approach coupled with prior literature information, differential network analysis [56] , [57] , [58] , [59] , [60] , [61] , [62] , [63] tools showed promise in identifying context-specific knowledge and highlighted genes and pathways for clinical impact [11] , [59] , [64] , [65] , [66] , [67] , [68] , [69] . While informative, the drawback of such “literature-first” data integration methods is that they only allow the study of known connections, which omits the substantial number of regulatory interactions not annotated in the literature [30] , [56] , [70] . Importantly, these approaches cannot identify novel interactions or associations in the datasets. Another group of data integration approaches are prior knowledge agnostic, which circumvents the limitations of literature-first methods [24] , [44] , [71] , [72] , [73] . These methods rely on extracting features from the input data and constructing models to discriminate between conditions. For instance, Zhang et al. used deep learning to integrate gene expression and copy number variance data from two different databases to identify distinct prognostic subtypes [24] . However, the trade-off of these methods is that they are more challenging to interpret because they lack direct incorporation of a biological structure (e.g., central dogma) into the data integration methodology and also do not take advantage of the wealth of available prior knowledge [11] , [74] , [75] . Despite progress, there remains a need for new tools and methods for biologically informed multi-omics integration without literature-driven pre-selection. Here, we introduce M ulti- O mics B inary I ntegration via L asso E nsembles (MOBILE) to integrate multi-omic datasets and identify context-specific interactions and pathways. Our approach does not eliminate data based on prior knowledge and also uses a well-established central dogma structure to aid biological interpretation. Robust associations are inferred between pairs of chromatin accessibility regions, mRNA expressions, and protein/phosphoprotein levels. By imposing this high-level structure, MOBILE is neither network structure agnostic (for better interpretability) nor heavily prior knowledge bound (for higher rates of novelty). We demonstrate the method using a recent multi-omic dataset generated by the NIH LINCS Consortium [76] . In that project, non-tumorigenic breast epithelial MCF10A cells were assayed for proteomic, transcriptomic, epigenomic, and phenotypic changes in response to six growth factor perturbations (EGF, HGF, OSM, IFNγ, TGFβ1, and BMP2; synapse.org/LINCS_MCF10A). We apply MOBILE to this dataset and obtain candidate context-specific associations. We then use these associations (i) to propose sub-networks of regulation for therapeutically important genes and (ii) to identify pathways preferentially activated by pairs of ligands from similar signaling families. First, MOBILE identifies regulatory mechanisms for IFNγ-controlled PD-L1 expression that have independent literature support. Secondly, MOBILE reveals–and independent experiments validate–that TGFβ1 but not BMP2 induces laminin pathway genes (especially laminin 5), causing stronger cell-to-cell and cell-to-surface adhesion through interactions with extracellular collagen, which leads to larger and more separated cells. Finally, we use MOBILE to explore breast cancer subtype-specific pathways by integrating patient-level transcriptomic and proteomic datasets from The Cancer Genome Atlas (TCGA) [1] . The biologically structured and data-driven MOBILE pipeline outlined here is widely applicable to integrate omics datasets for extracting context-specific network features and insights. A multi-omics LINCS perturbation dataset for integrative analysis The NIH LINCS Consortium recently released a unique and comprehensive multi-omics dataset (synapse.org/LINCS_MCF10A) that consists of molecular and phenotypic responses of MCF10A cells to multiple ligand perturbations over time [76] . Spanning a compendium of canonical receptor signaling classes, EGF, HGF, and OSM induced growth, while BMP2, IFNγ, and TGFβ1 inhibited growth. The cellular responses were measured using live-cell imaging, immunofluorescence (IF), and cyclic immunofluorescence [77] . The bulk molecular responses were assessed across five platforms. The proteomic assay was reverse phase protein array (RPPA [78] ), where specific phospho- or total protein levels were measured at 1, 4, 8, 24, and 48 h. The RNAseq transcriptomic dataset was single-end sequencing at 24 and 48 h. Chromatin accessibility was profiled by Assay for Transposase-Accessible Chromatin using sequencing (ATACseq), also at 24 and 48 h after stimulation. A pretreatment (T0 control) was quantified for all assay types. Overall, the MCF10A dataset provides an excellent template for applying the proposed data integration strategies, namely ATACseq, RNAseq, and RPPA as “big data” to be integrated, and the live-cell imaging / IF as assays informing associated cellular phenotypes. The MOBILE integrator We here integrated data from this LINCS dataset to identify context-specific pathways and regulatory mechanisms that control cellular phenotypes. The overall approach is summarized in Fig. 1 and presented in greater detail in Figs. 2 , 3 . The availability of epigenomic, transcriptomic, and proteomic datasets inspired a central-dogmatic view for data integration (Fig. 1 ). For compatibility across datasets and operability of the method, the MOBILE pipeline input included all three datasets with all ligands at 24 and 48 h only. Fig. 1: Multi-Omics Binary Integration via Lasso Ensembles (MOBILE) pipeline yields statistically robust, ligand-specific association networks. The MOBILE data integrator combines multi-omics, multi-assay datasets in a data-driven and central-dogmatic way. By leaving each ligand condition out from the input at a-time, the pipeline outputs robust ligand-specific association networks. These gene-level networks are used to infer differentially enriched pathways and to find regulatory sub-networks. Full size image Fig. 2: The MOBILE Integrator pipeline transforms input data into gene-level association networks. a The LINCS MCF10A datasets include proteomic (RPPA), transcriptomic (RNAseq), and epigenomic (ATACseq) assays. The number of analytes retained after data preprocessing are shown in parentheses on the y-axis. The heatmaps shown are the results from the hierarchical clustering of rows. Source data are provided as a Source Data file. b The Lasso module is used to integrate omics datasets one pair at a time. The associations between chromatin peaks (ATACseq) and mRNA levels (RNAseq) and between mRNA levels and protein levels (RPPA) are calculated separately. The two assay input matrices are structured to yield a Lasso coefficient matrix, which contains association coefficients between analytes of the two input matrices. Ten thousand instances of the Lasso matrices are generated. The coefficients that appear in at least half the matrices (>5000 times) are considered robust and the mean values of these coefficients populate the Robust Lasso Coefficient Matrix (RLCM). The non-zero elements in this matrix are called associations for the remainder of this work. c The Robust Lasso Coefficient Matrices of two input pairs are combined to generate Integrated Association Networks (IANs). These gene-level networks represent robustly, statistical associations inferred from multi-omics datasets, offering a new hypotheses generation tool to look for ligand or gene-set specific sub-networks. Node colors represent; blue:RNAseq, purple:ATACseq, and orange:RPPA, and the edge widths correlate with the magnitude of the association coefficients. Full size image Fig. 3: The leave-one-group-out (LOGO) module generates ligand-specific association networks. We employed a leave-one-group-out (LOGO) analysis to find associations associated with exclusion/inclusion of that specific condition. We excluded one set of ligand conditions (24 and 48 h) from the input matrices, ran the Lasso module (Fig. 2b ) with a smaller number of columns, and obtained a new Robust Lasso Coefficient Matrix, named ligand-specific coefficient matrices. Comparing the resulting matrix from the LOGO module to the FULL-data Lasso coefficient matrix, we determined the “ligand-dependent” coefficients (ones that appear only in LOGO IAN and coefficients that are present only in FULL-data IAN) to create the final ligand-specific associations list. Repeating the process for each ligand treatment condition, we obtained six ligand-LOGO IANs. Full size image Following the central dogma that information flows from DNA to RNA to protein, we paired ATACseq-RNAseq and RNAseq-RPPA matrices. First, we calculated robust and parsimonious statistical associations between features of input data (Fig. 2a , see Methods) using replicated penalized regression models (Fig. 2b and Supplementary Data 1, 2 ). We applied Lasso (least absolute shrinkage and selection operator [37] , [79] ) regression to infer sets of sparse matrices that can be interpreted as statistical networks connecting biochemical species, such as mRNAs, chromatin peaks, or total protein and phosphorylation levels. The repetitive application of Lasso, called the Lasso module, yielded an ensemble of matrices, from which we picked one as the robust associations matrix. When we used all the ligand conditions from the LINCS dataset as input, the Lasso module output is called the FULL-data matrix. To finalize the data integration and generate data-driven networks, we merged the robust associations matrices obtained from RPPA+RNAseq and RNAseq+ATACseq input pairs into an Integrated Association Network (IAN) (Fig. 2c ). The IANs are coalesced gene-level networks, where nodes represent genes of the assay analytes (genes from input matrix rows) and edges represent robust Lasso coefficients calculated between the analyte levels (Supplementary Fig. 1 ). We then systematically excluded different ligand conditions (both 24- and 48-h data) from the training input and ran the LOGO (leave-one-group-out) module (Fig. 3 ). The input data with a smaller number of columns were then processed via a regular Lasso module (Fig. 2b, c ), and new Robust Lasso Coefficient Matrices were generated. Next, by comparing the FULL-data associations matrix to the newly inferred LOGO-condition associations matrix, we identified associations dependent on the exclusion/inclusion of that specific condition’s data. This “ligand”-specific association list is used to create the ligand-LOGO-IAN. Repeating the process for each ligand condition in the dataset, we obtained six ligand-specific IANs (Fig. 3 ). We hypothesized that the robust associations that change as a result of this LOGO analysis will have information regarding the context-specificity of the left-out ligand condition. The ligand-specific IANs, together with the FULL IAN were the major data-integration products of the MOBILE. Comparison of pairs of ligand IANs nominated differentially activated networks and ligand-specific regulatory mechanisms spanning DNA states to protein levels. To facilitate biological interpretation, we performed gene-set enrichment analysis (GSEA [80] ) using the Reactome database [81] that enabled us to identify pathways linked to ligand-specific IANs. We then nominated ligand-specific pathways and novel edges associated with distinct phenotypes observed in the image data. MOBILE identifies known biology We investigated the robustness of the MOBILE predictions by performing a gene-set enrichment analysis (GSEA) for pathways using the FULL and ligand-specific integrated associations networks (IANs) and asking whether our approach can capture canonical biological observations. First, we identified ligand-dependent association lists by comparing each ligand IAN to the FULL IAN. Next, these association lists were coalesced into gene-level networks and the nodes were ranked based on the sum of edge weights (association magnitudes) of that node (Supplementary Data 3 ). We ran GSEA on these eight (FULL, PBS, EGF, HGF, OSM, IFNG*, BMP2*, and TGFB1*) pre-ranked gene-lists and found that the top enriched pathways were cell cycle in all conditions ( p < 0.05 and FDR <0.1, Fig. 4a and Supplementary Data 4 ). Indeed, eight of the top 15 pathway enrichments across conditions are cell cycle-related, affirming the fact that the LINCS dataset was generated using combinations of pro/anti-growth factors and cells continue to grow after all perturbations (Supplementary Fig. 2 and Supplementary Data 5 ). Fig. 4: MOBILE inferred IANs are enriched for canonical pathways and the top associations are literature-verified interactions. a Gene set enrichment analysis using genes of ligand-dependent associations revealed cell cycle, interferon, and cytokine signaling pathways. Only the top ten significantly enriched pathways are shown for each ligand perturbation ( p values <0.05, FDR <0.1, significance tested using default GSEA settings of single-tail null distributions [80] ). The bar height corresponds to the normalized enrichment scores (NES). Stars denote pathways enriched specifically for the corresponding ligand condition when only considering the top ten pathways shown. Asterisk denotes conditions with additional EGF treatment. Source data are provided as a Source Data file. b MOBILE finds known and novel associations between proteins, transcripts, and chromosomal region genes. The top ten magnitude-wise associations between RPPA-RNAseq and RNAseq-ATACseq of the FULL IAN are presented. More than half of the associations have prior literature evidence, while some are “Self” associations of the same gene in different assays. Two associations include non-annotated gene products labeled as “Unknown”. At least four of the associations are “Novel” predictions of the MOBILE pipeline. ~ denotes references not showing a direct (causative) relationship between the genes but co-mentioning them as biomarkers of different cancer subtypes or with relationships of candidates’ isoforms. The MOBILE inferred association values are between −1 and 1. Full size image Other highly enriched pathways in the HGF dependent gene-list were Rho GTPase related (Fig. 4a ). It was shown before that Rho GTPase activity is required for HGF-induced cell scattering [82] . OSM-dependent pathway enrichments included cytokine/interleukin and ECM pathways (Fig. 4a ). The top four highly enriched pathways of IFNG* condition were interferon signaling, in line with the fact that IFNγ had a strong signal in the LINCS dataset [76] . BMP2-dependent top pathways were ECM, interferon, and interleukin related in addition to the cell cycle. Finally, the TGFB1* condition had transcriptional and DNA regulatory pathways enriched (Fig. 4a ). These observations confirmed that our approach can recover known biology and also that it can extract meaningful ligand-specific associations. Next, we asked whether MOBILE-inferred associations (edges) are consistent with prior knowledge. The highest magnitude associations of the FULL analysis are the most robust across all perturbations and time points (Fig. 4b , Supplementary Data 1, 2 ). Among them, the top candidate interaction is the connection between PPFIA4 (Protein Tyrosine Phosphatase Receptor Type F Polypeptide-Interacting Protein Alpha-4) and HIF1A (Hypoxia Inducible Factor 1 Subunit Alpha). The PPFIA4 gene was shown to be upregulated in response to hypoxia (through HIF1 ) in all types of breast cancer cell lines and normal-like epithelial cells, including MCF10A [83] . The highest association between ATACseq and RNAseq data is the SLC2A1 (Solute Carrier Family 2 Member 1) and CASP14 (Caspase 14). Interestingly, these two genes were also part of the hypoxia-induced genes list [83] . There exists literature evidence for the other highest-ranking associations (Fig. 4b ). Some were (i) shown to be part of prognostic markers ( SLC12A4 - CHEK2 [84] ), (ii) differentially expressed together in response to perturbations ( SEMA3C - TCEAL1 [85] , IGFBP2 - SIX1 [86] , TINCR - POU2AF1 [87] , NTSR1 - TOMM6 [88] ), and (iii) part of gene signatures for different classes of tumors ( SNORA73A - MAPK [89] , FDCSP - GJA1 [90] ). A few of the associations had related mechanistic interactions as well (CDC42-MTOR [91] , [92] , IGFBP2-SIX1 [86] , WTAP-STAT3 [93] , [94] , TINCR-POU2AF1 [87] ). The remaining associations are either Self: same gene, different data type, Unknown: non-curated gene(s), or Novel: no known interactions to the best of our knowledge. These pieces of information from the literature, in part, verify that the MOBILE inferred associations have biological meaning. Identification of associations between IFNγ stimulation and PD-L1 regulation After establishing that MOBILE can recapitulate known biological interactions, we asked whether it could identify regulatory mechanisms within a single IAN. We focused on IFNγ, which had a strong signal in the LINCS dataset [76] and is a critical part of the immune response within the tumor microenvironment [95] , [96] . The cytokines within the environment, especially IFNγ, can induce transient PD-L1 (gene name: CD274 ) expression (Fig. 5a ) [97] , [98] , [99] , [100] . PD-L1 is a transmembrane protein that binds to its receptor PD-1 expressed in T cells and inhibits immunological tumor clearance. Both PD-L1 and PD-1 belong to a class of so-called “checkpoint” proteins; [98] , [101] immune checkpoint inhibitors are a new class of immunotherapeutic anti-cancer drugs [100] , [102] . However, PD-L1 expression is not correlated with patient response and is highly variable depending on tumor stage, site, and type. Consequently, predicting tumor responses to PD-1/PD-L1 blockade remains a challenge, and better biomarkers are needed to stratify patients. Therefore, an in-depth understanding of the regulatory mechanism of PD-L1 expression is still needed to provide new immunotherapeutic insights and potentially identify new drugs [103] . To investigate this question, we decided to explore sub-networks between IFNγ signaling and PD-L1 expression within the data-driven IFNγ integrated associations network. Fig. 5: Exploration of a single integrated association network reveals new links between IFNγ signaling and PD-L1. a IFNγ secreted by T cells induces PD-L1 expression through JAK/STAT/IRF1 and other canonical pathways (black arrows). The PD-L1 on the cell surface then interacts with PD-1 on the immune cells to induce tumor cell death. However, the PD-1/PD-L1 therapy yields inter- and intratumor heterogeneous responses, and there is a need to identify new non-canonical targets (represented by red arrows). b The IFNγ induces IRF1 and PD-L1 production in MCF10A cells. Data shown are from three independent biological replicates and error bars represent the standard error of the mean. Source data are provided as a Source Data file. c The IFNG associations' network (IFNγ-IAN) is a data-driven large-scale network of connections. The associations are coalesced into gene-level nodes, and associations with greater than 0.01 absolute value are shown. d The sub-network of the IFNγ – PD-L1 relationship is significantly smaller than the IFNγ-IAN. The sub-network is generated by filtering for 14 genes and has seven hubs (PD-L1 ( CD274 ), IFNGR1 , IRF1 , IRF9 , JAK2 , STAT1 , STAT3 ) connected to 290 other genes. Node colors represent; blue:RNAseq, purple:ATACseq, and orange:RPPA and the edge widths correlate with the magnitude of the association coefficients. e A closer look at the connections between IRF1 and PD-L1 ( CD274 ) genes shows a breadth of different functional genes. f Compared to no or EGF-only stimulation, the connecter genes are upregulated (RNAseq) in IFNγ stimulated condition. Additionally, the ACSL5 peak is more accessible similar to the canonical IFNγ downstream genes (ATACseq). The data shown are the average values from three independent biological replicates. Source data are provided as a Source Data file. Full size image In the LINCS dataset, IFNγ was tested in combination with EGF, so we isolated the IFNγ response by comparing the IFNγ condition (IFNγ + EGF) to EGF-only samples. We confirmed that IFNγ stimulation uniquely upregulated canonical downstream elements, including IRF1, interferon regulatory factor, and PD-L1 ( CD274 gene) (Fig. 5b ). Next, we identified a set of nine genes ( IFNG , IFNGR1 , IFNGR2 , STAT1 , STAT3 , JAK1 , JAK2 , IRF1 , and IRF9 ) from the canonical IFNγ pathway (REACTOME R-HSA-877300) and filtered the connections of the genes together with PD-L1 ( CD274 ) and PD-1 ( CD279 ) from IFNG-IAN (Fig. 5c ). The resulting sub-network had 297 nodes and 321 edges (Fig. 5d and Supplementary Data 6, 7 ). The hubs in that sub-network were from the input gene-list, including IRF1 , STAT1 , STAT3 , and CD274 (PD-L1). We examined the connections between IRF1 and PD-L1 (Fig. 5e ) and identified five nodes: BST2 , CLIC2 , FAM83D , ACSL5 , and HIST2H2AA3 . The mRNA levels of these five genes were elevated in the IFNγ + EGF condition compared to EGF-only samples (Fig. 5f ). Of the five genes, three had strong literature support. BST2 was recently shown to be part of a gene signature for anti-CTLA4 response in melanoma [104] . CLIC2 is co-expressed with PD-L1/PD-1 in breast cancer and is a biomarker candidate for favorable prognosis [105] . And although not directly linked to IFNγ/PD-L1 axis, FAM83D was shown to regulate cell growth and proliferation and was implicated as a prognostic marker in breast and gastric cancers [106] , [107] , [108] . Moreover, its FAM83A isoform was shown to affect PD-L1 expression [109] . We could not find any literature data for two genes ( ACSL5 and HIST2H2AA3 ) and their relationships to IFNγ and PD-L1 function, suggesting potentially novel diagnostic or therapeutic targets for immunotherapy. Importantly, the concordance of some findings with recent literature reinforces the notion that MOBILE-based nomination of interactions has biological value. TGF-β superfamily members TGFβ1 and BMP2 induce different morphological phenotypes via collagen-laminin signaling Both BMP2 and TGFβ1 are members of the TGF-β superfamily and share most downstream pathways, including canonical SMAD signaling [110] , [111] . Both ligands induce cell differentiation and show anti-growth/anti-proliferative effects, whereas SMAD signaling shows immense versatility and specificity, mostly affected by the cross-talk mechanisms and the cellular context [110] , [111] , [112] , [113] , [114] , [115] , [116] , [117] , [118] . Imaging data of cells grown on collagen-coated culture plates from LINCS [76] indicated that BMP2 induces a significantly higher number of cells in clusters as compared to that induced by TGFβ1 (Fig. 6a, top ). Correspondingly, TGFβ1 induced morphologically larger cells [119] , [120] that occupy more surface area (Fig. 6a, bottom ). We used the ligand-specific IANs (Supplementary Fig. 3 ) and subsequent pathway enrichment analyses to find non-canonical mechanisms that underly the differential phenotypes caused by these two highly similar ligands. We ranked the nodes of the TGFβ1 and BMP2 IANs (Supplementary Data 8, 9 ) based on the sum of edge weights entering that node (Supplementary Data 10 , 11 ) and ran GSEA on these pre-ranked gene-lists [80] , [121] . We then looked for curated Reactome pathways [81] significantly enriched ( p < 0.05 and FDR <0.1) in either gene-list (TGFβ1 or BMP2 IAN genes) (Fig. 6b ). Seven of the enriched pathways under BMP2 and TGFβ1 treatment conditions are shared (Fig. 6c gray circles, and Supplementary Data 12, 13 ). The shared pathways are all cell cycle and proliferation-related. Multiple pathways are specific to a single condition (Fig. 6b , BMP2: purple and TGFβ1: gold). BMP2-enriched pathways include DNA regulation and G1/S transition. The TGFβ1-only group has DNA damage and ECM regulation-related clusters of pathways. It is important to note that pathway enrichment analyses on shuffled data-derived TGFβ1 and BMP2-specific IANs did not yield any pathways ( p value <0.05, and FDR <0.1). Fig. 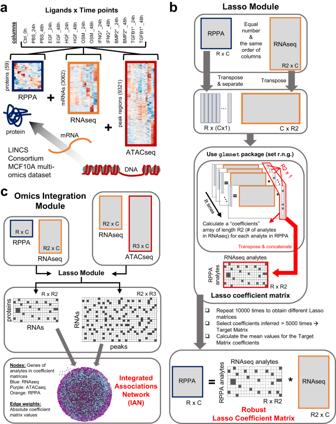Fig. 2: The MOBILE Integrator pipeline transforms input data into gene-level association networks. aThe LINCS MCF10A datasets include proteomic (RPPA), transcriptomic (RNAseq), and epigenomic (ATACseq) assays. The number of analytes retained after data preprocessing are shown in parentheses on the y-axis. The heatmaps shown are the results from the hierarchical clustering of rows. Source data are provided as a Source Data file.bThe Lasso module is used to integrate omics datasets one pair at a time. The associations between chromatin peaks (ATACseq) and mRNA levels (RNAseq) and between mRNA levels and protein levels (RPPA) are calculated separately. The two assay input matrices are structured to yield a Lasso coefficient matrix, which contains association coefficients between analytes of the two input matrices. Ten thousand instances of the Lasso matrices are generated. The coefficients that appear in at least half the matrices (>5000 times) are considered robust and the mean values of these coefficients populate the Robust Lasso Coefficient Matrix (RLCM). The non-zero elements in this matrix are called associations for the remainder of this work.cThe Robust Lasso Coefficient Matrices of two input pairs are combined to generate Integrated Association Networks (IANs). These gene-level networks represent robustly, statistical associations inferred from multi-omics datasets, offering a new hypotheses generation tool to look for ligand or gene-set specific sub-networks. Node colors represent; blue:RNAseq, purple:ATACseq, and orange:RPPA, and the edge widths correlate with the magnitude of the association coefficients. 6: TGFβ1 and BMP2 induce different morphological phenotypes by differentially activating collagen-laminin signaling. a TGFβ1 and BMP2 induce phenotypically different responses at 48 h after ligand treatment [76] . Representative images are adapted examples from eight biological replicates. b Both TGFβ1 and BMP2 networks are enriched in cell cycle and proliferation-related pathways (gray circles). TGFβ1 alone is shown to regulate ECM-related pathways, whereas BMP2 network genes are linked to other membrane receptor-related signaling pathways and cell cycle checkpoints. Node size is proportional to the enrichment scores and edge widths represent the number of overlapping genes. c The expression levels of the laminin pathway genes (left) are upregulated by TGFβ1. The chromosomal regions (peaks, right panel) of the laminin genes are more accessible in the TGFβ1 condition. Transcriptomic and epigenomic data shown are the average values from three independent biological replicates. Source data are provided as Source Data file. d BMP2 (purple) and TGFβ1 (gold) induce similar anti-growth responses but yield different microenvironmental and spatial characteristics. Both ligands inhibit cell proliferation (well cell counts, shaded region). BMP2 induces a larger number of cells in clusters compared to TGFβ1 (cells per cluster, shaded region, p value = 0.0175). TGFβ1 causes cells to spread and have a longer distance to their second nearest neighbors (distance to second neighbors, shaded region, p value = 9.4032E-06). Cells grown in non-collagen-coated regular tissue-culture plates show phenotype reversal of cells per cluster and distance-to-second-neighbor metrics (unshaded regions, middle and right box plots), with no significant cell number differences between BMP2 and TGFβ1. The box edges correspond to the 25th−75th percentiles, the horizontal black lines represent the median, and the dots are individual data points. The whiskers extend to the non-outlier extremes. ns: not significant, asterisk: p value <0.05, three asterisks: p value <0.001. Significance using two-sided Student’s t -test with unequal variance. Data shown are from N = 6, 6, 8, and 4 biological replicates respectively. Source data are provided as Source Data file. e The schematic of TGFβ1 specific regulation of a non-SMAD pathway, inferred by the MOBILE pipeline. TGFβ1 induces laminin pathway gene expression and leads to cell scattering and cell spreading with larger cells, when compared to BMP2 stimulation. Full size image The laminin interactions (REACTOME R-HSA-3000157) is among the TGFβ1-only enriched pathways. Laminins are a family of proteins that regulate cell-to-cell and cell-to-matrix interactions [122] , [123] , [124] , [125] , [126] , [127] , by binding to collagen [128] and integrin receptors [129] . Depletion of ECM laminin or collagen disrupts cellular attachment [122] , [130] . Differential regulation of these processes might offer a candidate mechanism for the observed TGFβ1 and BMP2 phenotypic difference: only TGFβ1 induces laminin gene expression that then interacts with the collagen-coating of the culture plate, which induces tighter cell-to-cell and cell-to-ECM interactions leading to more spreading and stretching cells. So, we analyzed the activity of the laminin pathway under TGFβ1 and BMP2 stimulation by comparing the mRNA levels (the MOBILE input data) of the pathway genes (Fig. 6c ). The mRNA levels of laminin, collagen, and integrin subunits were elevated at 24 and 48 h (Fig. 6c , left), and corresponding transcription binding sites were more accessible in TGFβ1 stimulated cells (Fig. 6c , ATACseq data, right). In the LINCS dataset, cells were cultured and treated on collagen-coated plates [76] and both ligands inhibited cell proliferation as compared to EGF-only control (Fig. 6d , left panel). Additionally, BMP2 induced more cell clustering compared to TGFβ1 (Fig. 6d , middle panel), but TGFβ1 was shown to cause significantly larger distances to second nearest neighbors (Fig. 6d , right panel). To test the hypothesis that TGFβ1-specific phenotypes depend on activation of laminin-collagen (in ECM) interactions (Fig. 6e ), we cultured cells on non-collagen-coated plates and stimulated them with TGFβ1 or BMP2 (+EGF, as done in the LINCS dataset [76] ). Removal of the collagen caused a reversal of the TGFβ1-induced phenotype. The number of cells per cluster and distance to the second nearest neighbors are similar in BMP2 and TGFβ1 stimulated cells in the absence of collagen-coating (Fig. 6d , middle and right panels). Overall, these analyses confirmed that MOBILE identified a context-specific network that explains differential phenotype between two highly similar ligands. Finally, although MOBILE analysis identified the laminin pathway as potentially explanatory for differential phenotype, we wondered whether such a conclusion could be reached by standard differential expression analysis. Considering the same list of pre-filtered 3062 transcripts that were input to the MOBILE pipeline, we determined BMP2 or TGFβ1 up and downregulated genes at 24- or 48-h conditions. Next, we ranked the genes based on the fold-change (BMP2 vs TGFβ1 or TGFβ1 vs BMP2) and, similar to post-MOBILE enrichment analysis, we ran GSEA on these pre-ranked lists of genes (Supplementary Data 14 ). We then compared MOBILE results with the differential expression analysis results. The BMP2 upregulated, TGFβ1 upregulated, BMP2 downregulated, and TGFβ1 downregulated gene-lists alone did not yield any significant pathway enrichments ( p value <0.05 and FDR <0.1). However, we obtained a single significantly enriched pathway (REACTOME Extracellular Matrix Organization, R-HSA-1474244) when we looked at the combined list of TGFβ1 up- and down-regulated genes. The combined BMP2 regulated gene-list yielded 10 significantly enriched pathways, including ECM Organization (Supplementary Data 15 ), whereas the MOBILE pipeline yielded 39 (TGFβ1, Supplementary Data 12 ) and 20 (BMP2, Supplementary Data 13 ) enriched pathways using TGFβ1- and BMP2-specific IANs. This indicates that the MOBILE inferred ligand-specific association networks and their analyses extract more information about differential pathway enrichments as compared to standard methods. MOBILE infers subtype-specific and differentially activated pathways using paired-omics datasets from TCGA samples MOBILE is agnostic to data sources and can be applied to a variety of datasets when structured correctly. We show the applicability of the pipeline by using tumor transcriptomic (RNAseq) and proteomic (RPPA) data from the TCGA database [1] . In short, 878 samples were identified to have both transcript and protein data from the primary breast tumor site. Analysis of receptor expression was used to stratify these samples into clinically-relevant subtypes: 89 HER2-amplified (HER2-amp), 129 triple-negative (TNBC), and 308 estrogen and progesterone receptor positive (ER+/PR+) (see Methods and Supplementary Fig. 4 ). Following the MOBILE Lasso Module procedure (Fig. 2b ) and using all samples (878 cases), we generated a FULL breast cancer integrated association network (FULL-TCGA-IAN). Next, we calculated subtype-specific IANs with the LOGO module (Fig. 3 ). Then, the subtype IANs are pair-wise compared to each other and enriched Reactome pathways are determined (Fig. 7a , Supplementary Fig. 5 , and Supplementary Data 16 – 18 ). Specifically, the HER2-amplified subtype was enriched in membrane trafficking, lipid/steroid metabolism, and adaptive immune response-related pathways (Fig. 7a , purple and dark gray). In support of these observations, the literature data shows that HER2-amplified cell lines and tumor samples both have elevated FASN and ACAT1 function (fatty acid synthesis), leading to poor prognosis [131] , [132] , [133] , [134] and inhibitors to such targets enhance the efficacy of anti-HER2 therapies [135] . HER2-amplified cells were also shown to have high levels of endocytic and extracellular vesicle trafficking [136] . Fig. 7: MOBILE infers breast cancer subtype-specific and differentially activated pathways. a The LOGO-IANs are pair-wise compared and subtype-specific pathway enrichments are determined. The colors represent subtypes (purple: HER2-amplified, gold: TNBC, red: ER/PR-positive, gray: subtype shared), node size depends on pathway gene-set size, and edge width correlates with shared gene-set similarity of the connected nodes. Examples of pathways are labeled individually or as groups. b The pathways enriched in all LOGO-IAN conditions constitute the breast cancer (BRCA) core network. The list includes cell cycle, estrogen, MAPK, and PI3K signaling as well as transcriptional regulation and programmed cell death. Node size and edge width represent the gene-set size and gene-set similarity of the connected nodes, respectively. Full size image TNBC is a subtype with poor prognosis and aggressive phenotype. The MOBILE inferred TNBC-specific enriched pathways include receptor signaling pathways like Wnt and VEGF, keratinization, TCA cycle, and innate immune response-related pathways (Fig. 7a , gold and dark gray). In the literature, the TNBC subtype was shown to correlate with high VEGF activity and multiple antiangiogenic agents were included in combination therapies for aggressive tumors like TNBC [137] , [138] . Similarly, elevated and dysregulated Wnt signaling in TNBC was reported numerously [139] , [140] . In recent studies, suppression of the TCA cycle was shown effective in decreasing the growth and invasion of TNBC cells [141] , as increased TCA cycle utilization provides elevated ATP production for the cells [142] , [143] . Finally, the ER+/PR+ subtype was enriched in GPCR and aberrant PI3K signaling (together with TNBC), cell-cell communication, cellular senescence, and RUNX2-mediated transcription pathways (Fig. 7a , red and light gray). In the hormone receptor-positive subtype, hyper-activated PI3K activity was previously shown [144] , [145] , [146] , [147] . Moreover, cell-cell communication and signaling is elevated ER+ cell lines [148] , where chemotherapy-induced senescence is sensitive to hormone therapy [149] . Regarding RUNX2-mediated transcriptional activity, triple-positivity (ER+, PR+, RUNX2+) is prevalent, especially in grade 2 and 3 breast tumors [150] , with possible ER-RUNX2 mutual regulatory mechanisms [151] . Finally, G protein–coupled receptor superfamily, and especially the G-protein-coupled estrogen receptor (GPER) [152] , [153] , was shown to mediate estrogen-dependent kinase activity in breast cancer tumorigenesis and metastasis [154] , [155] , [156] . In addition to the subtype-specific enriched pathways, we summarized the common pathways enriched in all three subtypes (Fig. 7b and Supplementary Data 19 ). These include cell cycle, transcription, intracellular signaling, and programmed cell death pathways. Estrogen receptor (ESR)-mediated signaling was also included in the core network, most likely due to the facts that estrogen is critical and central in breast biology and the curated pathway gene-list coincides largely with major proliferation pathways (MAPK and PI3K) and transcription. Here we introduced the MOBILE pipeline to integrate and analyze multi-omics datasets in a data-driven way. Using a central-dogmatic framework, the method finds statistically robust integrated association networks (IANs) between pairs of epigenomic, transcriptomic, and proteomic analytes that are biologically interpretable. We explored context-specific IANs obtained via leave-one-group-out (LOGO) analysis, yielding (i) non-canonical connections with novel immunotherapeutic potential, (ii) differentially activated pathways to discriminate between highly similar ligand-receptor responses, and (iii) breast cancer subtype-specific pathway enrichments. The MOBILE pipeline can prioritize context-specific, differentially activated pathways and mechanisms. MOBILE identifies statistically significant associations, while LOGO analysis provides context-specificity. In our analysis of the LINCS MCF10A dataset, by holding out data from each ligand one at a time, associations that depend on the held-out data are inferred and cataloged as ligand-dependent. These ligand-dependent associations are the core of MOBILE integrator, enabling the exploration of single ligand-specific and differentially enriched pathways between multiple conditions. We expect that the exact method used for forming statistical associations (replicated Lasso) could be substituted with other methods [10] , [24] , [28] , [30] , [54] , [55] , [56] . However, by imposing matching time points, we miss time-lagged associations between mRNAs and proteins due to their temporal ordering. Thus, the next step for the MOBILE pipeline could be to become more flexible with respect to different time points for different assays to more fully exploit temporal dependence information for inference of associations. The above-mentioned matching column order for input matrices requirement of the MOBILE pipeline in this work does not restrict users to study only time points x ligand conditions. For instance, we applied MOBILE to TCGA datasets to infer cancer subtype-specific pathways, where the columns of input matrices were individual patients. Moreover, we previously showed that paired input data matrix pairs at different time points (rows: proteomic measurements, columns: different cell lines) could infer robust, time-dependent associations between proteins and phospho-proteins [37] . Another way to utilize the MOBILE pipeline is to find cell line-specific association networks by considering datasets like the Cancer Cell Line Encyclopedia (CCLE), where hundreds of cell lines were characterized with molecular and functional assays [2] , [157] . MOBILE could be set up where columns represent different cell lines, and the matrix pair are proteomic and transcriptomic data. By imposing different higher-level hierarchies for the MOBILE pipeline, researchers can explore different types of context-specificity by using data from either single or multiple assays. The current MOBILE pipeline is appropriate for use with continuous data only. This is partly due to the datasets we analyzed so far and in part due to the Lasso regression type selected. However, other methods within the glmnet package could be substituted, which would provide additional flexibility on the input data. Another limitation of the current framework is that input matrices need to be complete, without missing values; future versions of MOBILE could include data imputation methods to further enhance functionality and enable the use of sparse data. Nevertheless, the associations generated by MOBILE are all data-driven experimental candidates to study ligand-specific linkages between genes and gene products. The highest magnitude associations could suggest new hypotheses and inform the design of experiments to explore cross-talk mechanisms or unknown links in the literature. For instance, by analyzing the IFNγ-specific network only, we hypothesized new regulatory mechanisms of PD-L1, a critical immunotherapeutic target. Of the five MOBILE-hypothesized connector genes ( BST2 , CLIC2 , FAM83D , ACSL5 , and HIST2H2AA3 ) between IRF1 and PD-L1, BST2 was recently recognized as part of an immune/tumor-related signature that is significantly associated with the overall survival of skin cancer patients [104] . Specifically, the BST2 gene signature predicted a response to a CTLA4 antibody called ipilimumab, suggesting a mechanistic involvement in tumor progression. Secondly, CLIC2 was shown to be co-expressed with PD-L1 and PD-1 and act as a good prognosis marker with higher rates of tumor-infiltrating CD8 + T cells in breast cancer patients [105] . Finally, FAM83D was shown to be a potential oncogene with high expression levels associated with poor breast cancer prognosis [106] . Moreover, FAM83A (an isoform of FAM83D ) was shown to drive PD-L1 expression and be correlated with poor lung cancer prognosis [109] . These results suggest that context-specific gene-gene associations identified through MOBILE are potential biomarkers for prognosis and patient response to immune checkpoint inhibition. Another key capability of the MOBILE pipeline is the IAN-comparative analysis. For instance, we hypothesized and then experimentally validated that the phenotypic differences between TGFβ1 and BMP2 perturbations are caused by cell-ECM interactions, specifically laminin-collagen. When we assessed responses in the absence of collagen-coating, the two ligands induced similar changes, in agreement with prior findings that both TGFβ1 and BMP2 induce cell differentiation, inhibit cell proliferation, and signal through similar canonical pathways [111] , [112] , [113] . Additionally, it was shown before that laminin/collagen pathway inhibition leads to cell-ECM attachment disruption [122] , [130] . However, there are other TGFβ1-specific ECM-related pathways (Fig. 6b ) and genes that could be further explored for differences between BMP2 and TGFβ1 conditions. Similarly, studying other ligand-IAN pairs (e.g., EGF vs HGF, IFNγ vs TGFβ1, and OSM vs IFNγ) could suggest additional data-driven hypotheses. We also demonstrated that MOBILE performs well with patient data. By empirically defining three patient subtypes and applying LOGO, we determined association networks for HER2-amplified, triple-negative, and ER+/PR+ subtypes. The pair-wise comparison of corresponding IANs revealed subtype-specific and subtype-independent (core) enriched pathways. Most of the pathways were previously reported in association with the mentioned subtype, but MOBILE also provided hypotheses to explore further. An example of the latter is that the HER2-amplified subtype network was enriched for the adaptive immune response pathway, whereas the TNBC subtype was associated with innate immune response and keratinization pathways. Another next step would be to explore patient-specific IANs using the same TCGA input. The MOBILE pipeline here infers robust associations between genes and gene products without prior network knowledge input, enables the generation of context-specific, gene-level networks of different biological modalities in a data-driven way, and provides an exploration of these networks in a single or paired fashion to pinpoint differentially activated pathways. We believe the freely-available MOBILE pipeline will be broadly helpful in extracting context-specific insights from multi-omics datasets to help answer targeted biological questions. The Lasso module The multi-omics datasets from the LINCS consortium [76] are pre-processed using a raw variance filter to retain only 10% (RNAseq, ATACseq) and 20% (RPPA) highly variant analyte measurements across median summarized Level 4 data (Fig. 2a , synapse.org/LINCS_MCF10A, https://doi.org/10.6084/m9.figshare.20294229.v2 ). The variance cut-off provides that we only look at analytes with some variability across different (ligand and time point) conditions [158] , [159] , [160] . The difference in cutoff percentages is due to the difference in number of features across assays. RPPA had the least, thus retained at a higher percentage (20 compared to 10). The proteomic (RPPA), transcriptomic (RNAseq), and epigenetic (ATACseq) datasets are integrated with a central-dogmatic view, such that pairs of RPPA+RNAseq and RNAseq+ATACseq data matrices are run through the Lasso module (Fig. 2b, c ). The steps of the algorithm [37] are: 1. We use glmnet package for lasso regression [161] . The module takes two input matrices, Y =left hand side and X =right hand side, and our goal is to calculate matrix β in \({{{{{\bf{Y}}}}}}{{{{{\boldsymbol{=}}}}}}{{{{{\boldsymbol{\beta }}}}}}\cdot {{{{{\bf{X}}}}}}{{{{{\boldsymbol{+}}}}}}{{{{{\boldsymbol{\delta }}}}}}\) . The number and the ordering of columns in input matrices should be equal (Fig. 2b ). The rows are assay analytes measured and columns represent ligand/time point conditions. 2. The matrices are column-centered, row-centered, and row normalized. The preprocessing makes sure that the algorithm is not biased towards high-magnitude analyte measurements but focused on analyzing based on the shape of measurements across conditions. It also sustains that the offset value is moved toward zero. 3. We set the cross-validation parameter of glmnet package to 4 and turned off the input data standardization option. 4. Next, both matrices are transposed and the transposed Y matrix ( Y’ ) is separated into column vectors. 5. For each column k of the Y’ (or each row of input matrix Y ), a set of lasso regression coefficients are calculated using glmnet package. With every iteration, we obtain one row of the final coefficient matrix β and an offset value δ , which is negligible in this case (values less than 10 −7 ). We minimize the quantity: 
    ∑_i=1^C[Y_ki-∑_j=1^Rβ_kjX_ji-δ_k]^2+λ∑_j=1^R|β_kj|
 (1) 6. The λ factor (Eq. 1) is estimated via the inherent cross-validation step of the glmnet package. In short, a set of different λ values are tested, resulting in different sets of lasso coefficients, each with a potentially different number of non-zero coefficients. 7. We select the set of lasso coefficients (i.e., the lasso coefficient vector) corresponding to the minimum estimation error. 8. Repeating steps 5-7 as many times as the number of input Y rows, we obtain R-many Lasso coefficient vectors, each R2-long. 9. We concatenate the R-many R2-long vectors to obtain a Lasso coefficient matrix. 10. We repeat the (3–9) steps 10,000 times to obtain an ensemble of Lasso coefficient matrices. We start each estimation with a different seed for a random number generator. 11. We calculate the average value for every matrix position, based only on the matrices that are non-zero. We also find the coefficient indices (matrix positions) that appear (inferred as non-zero) at least half of the time (currently ≥5000 times). The overlap between these two matrices is called the Robust Lasso Coefficient Matrix (RLCM) and used for the rest of the analyses. 12. The final matrix ( β ) sustains the equality \({{{{{\bf{Y}}}}}}={{{{{\boldsymbol{\beta }}}}}}\cdot {{{{{\bf{X}}}}}}\) and contains association weights relating to the analyte levels of the two input matrices. 13. When the input data contains all experimental conditions, we named the resulting robust Lasso coefficient matrix as the FULL-data matrix. 14. We do steps 1-13 for (i) RPPA (matrix Y )-RNAseq (matrix X ) and (ii) RNAseq (matrix Y )-ATACseq (matrix X ) input data matrix pairs. 15. To show that the inferred coefficients are non-random, we repeated the above steps for sets of shuffled input matrices, using Matlab (R2018a and R2021b) randperm function. We saw that the randomized input matrices resulted in a significantly smaller number of coefficients inferred (Supplementary Fig. 6 ). We used the kstest2 function in Matlab to test for the significance in the differences (Kolmogorov-Smirnov distances) between real and shuffled conditions. We obtained p values = 0 for all comparisons, indicating that the real input has more information content and thus requires more coefficients to explain the data. The MOBILE simulation of RPPA-RNAseq inference takes around 2–3 s per run (10,000 instances are run in total: ~8 h), including the save function in a normal desktop/laptop. The RNAseq-ATACseq inference simulations were run on Clemson University Palmetto HPC and took around 8 h per 1000 iteration of the 10,000 instances (sources used per batch job: number of nodes = 1, number of CPUs = 40, memory = 360 gb). Ten batch jobs were run in parallel, and the results were concatenated offline afterward. The LOGO module In addition to the Lasso module, we employ the leave-one-group-out (LOGO) module (Fig. 3 ) to obtain a new robust Lasso coefficient matrix for each perturbation in the input dataset. Here, the perturbations are ligand combinations used. We create a ligand-specific matrix by excluding that ligand condition during the model run and comparing the resulting matrix to FULL-data robust Lasso coefficient matrix to determine the coefficients that depend on the existence of the corresponding ligand data. We apply the LOGO module for both RPPA-RNAseq and RNAseq-ATACseq input pairs. Similar in principle to cross-validation, the LOGO module here enabled us not just to integrate given datasets but to acquire ligand-specific associations. The integration When both proteomic-transcriptomic and transcriptomic-epigenetic robust Lasso coefficient matrices are obtained, they are merged into a single, gene-level network (Fig. 2c ). This network representation is named the Integrated Associations Network (IAN), where each node is a gene, and edge weights represent the Lasso coefficient magnitudes. Notably, the gene nodes can represent data from one or more RPPA, RNAseq, or ATACseq sets. Summarizing the networks at the gene level enabled us to explore pathway enrichments using GSEA [80] . GSEA and pathway enrichments Using the Lasso+LOGO modules and excluding one ligand condition at a time, we obtain seven LOGO IANs (PBS, EGF, HGF, OSM, IFNγ, TGFβ1, and BMP2) in addition to the FULL-data network. We compare each ligand network with the FULL-data network to determine ligand-dependent associations and create gene-level network visuals using Cytoscape [162] . Next, we calculate the weighted sum of edge weights for each gene node in the networks and rank them. Then, we run pathway enrichment analysis using GSEA [80] and Reactome to obtain a list of curated pathways enriched for each network (i.e., ligand-LOGO condition). We calculate the gene-level weight α for each gene k (Eq. 2 ) by summing over each edge width and normalizing by the total number of possible edges. α_gene_k=|∑_j=1^3062∑_i=1^59β_ij|_RPPA_RNAseq+|∑_j=1^3062∑_i=1^9321β_ij|_RNAseq_ATACseq/59· 3062· 9321
 (2) The ranked gene-lists are then imported into GSEA software (version 4.1.0) and used in the GSEAPreranked analysis. We select Reactome (v7.2) as the gene set database, keep the default 1000 permutations option, and keep the dataset as is without collapsing the gene symbols since we already use the HGNC identifiers. We also choose the classical weighting option and choose “149” as our seed for permutation for reproducibility. We repeat these steps for every ligand-specific ranked gene-list from the ligand-specific IANs. After the enrichment analysis successfully completes, we use the Enrichment Map Visualization tool of GSEA, together with Cytoscape (v3.7.1). We only retain pathways enriched with a p value less than 0.05 and a false discovery rate (FDR) of 0.1. The results for BMP2 and TGFβ1 are given in Supplementary Data 12 , 13 . For this comparison, we only retain coefficients with magnitudes larger than 0.1 (Supplementary Fig. 7 ). MOBILE performance on finding known interactions We determined the lists of genes represented in the RPPA-RNAseq and RNAseq-ATACseq input matrices and used them to obtain known (literature-based) interactions via stringApp [163] in Cytoscape [162] (Supplementary Data 20 , 21 ). Then, we counted the overlap between the literature interaction lists and 10,000 Lasso coefficient matrices of real (yellow distributions) and shuffled (orange and blue distributions) data (Supplementary Fig. 8 ). The real data derived Lasso matrices contained significantly more interactions “correctly” inferred in both RPPA-RNAseq and RNAseq-ATACseq cases. For the latter, the real data condition yielded twice the number of known interactions in post-selection shuffled data and almost twenty times the number of interactions inferred from pre-selection shuffled data. The number of known interactions identified by the Robust Lasso Coefficient Matrices are also counted and reported (dashed lines, Supplementary Fig. 8 ). TCGA data analysis TCGA breast cancer transcriptomic (RNAseq) and proteomic (RPPA) datasets are downloaded (accessed on November 12, 2022, Supplementary Data 22 ). A total of 1226 RNAseq and 919 RPPA data files were obtained, representing 1098 cases (or patients). The data are filtered for paired files per case with the primary tumor site only. The final list was comprised of 878 cases (data columns). Then, the datasets are further cleaned: (i) ribosomal nuclear, long noncoding, micro, and other unannotated RNA transcripts and transcripts measured only in less than 10% cases are excluded from RNAseq and (ii) measurements with NaN values in RPPA are removed. The finalized lists for the MOBILE pipeline contained 27,797 transcript levels (RNAseq) and 457 protein levels (RPPA). Next, three subtypes are determined using RNAseq measurements: (i) HER2-amplified (log2(HER2_fpkm+1) > 7), (ii) triple-negative (TNBC, log2(HER2_fpkm+1) < 7, log2(ER_fpkm+1) < 1, and log2(PR_fpkm+1) < 1), and (iii) estrogen and progesterone receptor positive (ER+/PR+, log2(HER2_fpkm+1) < 7, log2(ER_fpkm+1) > 3, and log2(PR_fpkm+1) > 3). About 89, 129, and 308 cases were selected for each subtype, respectively. Then, following MOBILE pipeline guidelines, only the top highly variant analytes (10% for RNAseq, 20% for RPPA) are retained. MOBILE Lasso Module (Fig. 2b ) is run using all samples (878 columns) to obtain the FULL-TCGA-IAN. By excluding sample columns for each subtype from the input data, we ran the LOGO module (Fig. 3 ) to obtain context-specific IANs. 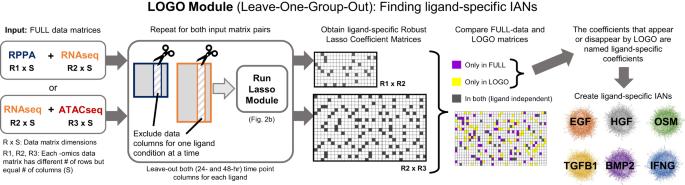Fig. 3: The leave-one-group-out (LOGO) module generates ligand-specific association networks. We employed a leave-one-group-out (LOGO) analysis to find associations associated with exclusion/inclusion of that specific condition. We excluded one set of ligand conditions (24 and 48 h) from the input matrices, ran the Lasso module (Fig.2b) with a smaller number of columns, and obtained a new Robust Lasso Coefficient Matrix, named ligand-specific coefficient matrices. Comparing the resulting matrix from the LOGO module to the FULL-data Lasso coefficient matrix, we determined the “ligand-dependent” coefficients (ones that appear only in LOGO IAN and coefficients that are present only in FULL-data IAN) to create the final ligand-specific associations list. Repeating the process for each ligand treatment condition, we obtained six ligand-LOGO IANs. Finally, the subtype-LOGO-IANs are pair-wise compared to each other, and enriched pathways are determined. Cell culture MCF10A cells (ATCC #CRL-10317, acquired from LINCS Consortium/Gordon Mills and STR verified internally in March 2019) are cultured in DMEM/F12 (Gibco #11330032) medium supplemented with 5% (by volume) horse serum (Gibco #16050122), 20 ng/mL EGF (PeproTech #AF-100-15), 0.5 mg/mL hydrocortisone (Sigma #H-0888), 10 μg/mL insulin (Sigma #I-1882), 100 ng/mL cholera toxin (Sigma #C-8052), and 2mM l -Glutamine (Corning #25-005-CI). Cells were cultured at 37 o C in 5% CO 2 in a humidified incubator and passaged every 2–3 days with 0.25% trypsin (Corning #25-053-CI) to maintain subconfluency. Experimental starvation medium is DMEM/F12 medium supplemented with 5% (by volume) horse serum (Gibco #16050122), 0.5 mg/mL hydrocortisone (Sigma #H-0888), 100 ng/mL cholera toxin (Sigma #C-8052), and 2 mM l -glutamine (Corning #25-005-CI). Mycoplasma testing The cells were tested for Mycoplasma using a detection kit (Lonza #LT07-701). Following the manufacturer protocol, growth media (2 mL) from the culture plate was spun at 200× g for 5 min, and 100 μL from the cleared supernatant was transferred into a well of a 96-well plate. About 100 μL testing Reagent was added into the same well and let settle for 5 min. Then luminescence is measured in Synergy H1 microplate reader (Agilent Technologies, Inc., CA, USA) with Gen5 (v3.08) software. The Gain was set to 200, the integration time to 1 s, and a single reading was captured. Then, the plate is returned under the hood and 100 μL of testing Substrate was added into the same well. The plate was left to settle for 10 min at room temperature. Then, the second luminescence reading (cell supernatant, Reagent, and Substrate) was taken with the same parameters. A ratio of less than 1 indicates a negative test. Validation experiments The cells were seeded in full growth media at 2000 cells/well in tissue culture treated (no collagen-coating) 96-well plates (Falcon #353072). After loading, plates were left to settle under the hood for 30 min and then placed in the incubator for 10 h. Next, the media is exchanged for experimental starvation media for 15 h. Then, media are replaced with fresh, experimental media containing the ligand(s): EGF (10 ng/mL, R&D Systems #236-EG), BMP2 (20 ng/ml, R&D Systems #355-BM) + EGF (10 ng/ml), and TGFβ1 (10 ng/ml, R&D Systems #240-B) + EGF (10 ng/ml). Each condition was repeated in triplicate. The plates are incubated for ~48 h. The cells are fixed using %2 paraformaldehyde (Alfa Aesar #43368) and stained with Hoechst (1:10000, by volume, BD Biosciences #561908) for nucleus localization. The plate was left for 1 h at room temperature. The wells are washed once with 1X PBS and replenished with 40 μl/well PBS. Imaging The plates are imaged at 10X magnification with phase contrast objective (Agilent/BioTek part number 1320516) and TagBFP filer cube (Agilent/BioTek part number 1225115, excitation 390 nm, emission 447 nm). A total of 10 × 8 fields of view per well? are imaged with laser autofocus on the Cytation5 (Agilent Technologies, Inc., CA, USA). When reading was done, the tiles were montaged together by the Gen5 (v3.04, Agilen/BioTeK) software using phase contrast images as registration template (fusion method = linear blend, final image reduction to 13.71%). The imaging parameters for phase contrast were LED = 10, Integration time = 8, and Gain = 24. The parameters for the TagBFP channel were LED = 10, Integration time = 36, and Gain = 24. Image processing and quantification The images are processed for cell segmentation and finding cell centroids. In short, TrackMate (v7.1.0) plugin from ImageJ (v2.3.0/1.53 f) is used to locate cell nuclei in each image (Hoechst stain + BFP channel, see https://doi.org/10.6084/m9.figshare.20294229.v2 ) and the summary was exported as a comma separated file (see https://doi.org/10.6084/m9.figshare.20294229.v2 ). The parameters for the plugin were Detector=LoG, Estimated object diameter=5 pixels, Quality threshold=0, Pre-process with median filter=ON, Sub-pixel localization=ON, and Initial thresholding=Auto. Spatial and microenvironmental metric calculations The csv files exported by ImageJ included each cell object as a row and reported its center coordinates with other default information. 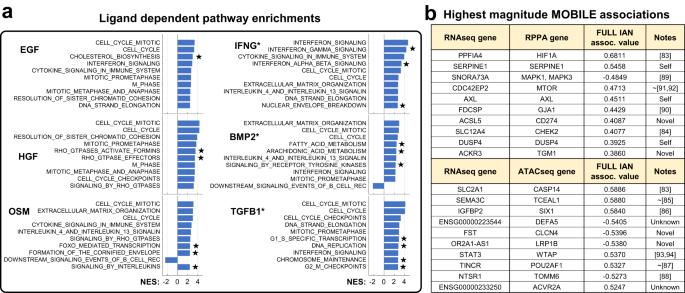Fig. 4: MOBILE inferred IANs are enriched for canonical pathways and the top associations are literature-verified interactions. aGene set enrichment analysis using genes of ligand-dependent associations revealed cell cycle, interferon, and cytokine signaling pathways. Only the top ten significantly enriched pathways are shown for each ligand perturbation (pvalues <0.05, FDR <0.1, significance tested using default GSEA settings of single-tail null distributions80). The bar height corresponds to the normalized enrichment scores (NES). Stars denote pathways enriched specifically for the corresponding ligand condition when only considering the top ten pathways shown. Asterisk denotes conditions with additional EGF treatment. Source data are provided as a Source Data file.bMOBILE finds known and novel associations between proteins, transcripts, and chromosomal region genes. The top ten magnitude-wise associations between RPPA-RNAseq and RNAseq-ATACseq of the FULL IAN are presented. More than half of the associations have prior literature evidence, while some are “Self” associations of the same gene in different assays. Two associations include non-annotated gene products labeled as “Unknown”. At least four of the associations are “Novel” predictions of the MOBILE pipeline. ~ denotes references not showing a direct (causative) relationship between the genes but co-mentioning them as biomarkers of different cancer subtypes or with relationships of candidates’ isoforms. The MOBILE inferred association values are between −1 and 1. The files were imported, and the cells per cluster and distance-to-neighbors metrics were evaluated using R (v4.1.3) scripts (on figshare https://doi.org/10.6084/m9.figshare.20294229.v2 , github.com/cerdem12/MOBILE) and packages (readr v2.1.2, dplyr v1.0.9, ggplot2 v3.3.5, tidyr v1.2.0, stringr v1.4.0, LPCM v0.46-7, foreach v.1.5.2) and RStudio (2022.02.0 + 443 Prairie Trillium release). 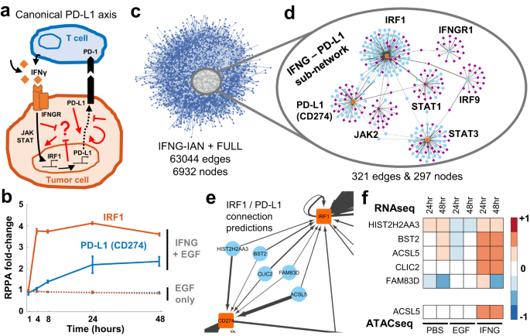Fig. 5: Exploration of a single integrated association network reveals new links between IFNγ signaling and PD-L1. aIFNγ secreted by T cells induces PD-L1 expression through JAK/STAT/IRF1 and other canonical pathways (black arrows). The PD-L1 on the cell surface then interacts with PD-1 on the immune cells to induce tumor cell death. However, the PD-1/PD-L1 therapy yields inter- and intratumor heterogeneous responses, and there is a need to identify new non-canonical targets (represented by red arrows).bThe IFNγ induces IRF1 and PD-L1 production in MCF10A cells. Data shown are from three independent biological replicates and error bars represent the standard error of the mean. Source data are provided as a Source Data file.cThe IFNG associations' network (IFNγ-IAN) is a data-driven large-scale network of connections. The associations are coalesced into gene-level nodes, and associations with greater than 0.01 absolute value are shown.dThe sub-network of the IFNγ – PD-L1 relationship is significantly smaller than the IFNγ-IAN. The sub-network is generated by filtering for 14 genes and has seven hubs (PD-L1 (CD274),IFNGR1,IRF1,IRF9,JAK2,STAT1,STAT3) connected to 290 other genes. Node colors represent; blue:RNAseq, purple:ATACseq, and orange:RPPA and the edge widths correlate with the magnitude of the association coefficients.eA closer look at the connections betweenIRF1and PD-L1 (CD274) genes shows a breadth of different functional genes.fCompared to no or EGF-only stimulation, the connecter genes are upregulated (RNAseq) in IFNγ stimulated condition. Additionally, theACSL5peak is more accessible similar to the canonical IFNγ downstream genes (ATACseq). The data shown are the average values from three independent biological replicates. Source data are provided as a Source Data file. The script is adapted from github.com/MEP-LINCS/MDD/blob/master/R/MDD_Immunofluorescence_Lvl0Data_Processing.R [76] . Statistics and reproducibility Although no statistical method was used to predetermine sample sizes, community standards were followed, and at least three biological replicates were run. 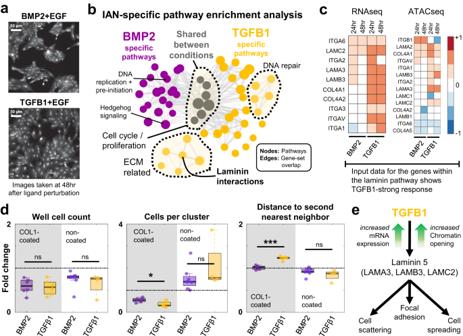Fig. 6: TGFβ1 and BMP2 induce different morphological phenotypes by differentially activating collagen-laminin signaling. aTGFβ1 and BMP2 induce phenotypically different responses at 48 h after ligand treatment76. Representative images are adapted examples from eight biological replicates.bBoth TGFβ1 and BMP2 networks are enriched in cell cycle and proliferation-related pathways (gray circles). TGFβ1 alone is shown to regulate ECM-related pathways, whereas BMP2 network genes are linked to other membrane receptor-related signaling pathways and cell cycle checkpoints. Node size is proportional to the enrichment scores and edge widths represent the number of overlapping genes.cThe expression levels of the laminin pathway genes (left) are upregulated by TGFβ1. The chromosomal regions (peaks, right panel) of the laminin genes are more accessible in the TGFβ1 condition. Transcriptomic and epigenomic data shown are the average values from three independent biological replicates. Source data are provided as Source Data file.dBMP2 (purple) and TGFβ1 (gold) induce similar anti-growth responses but yield different microenvironmental and spatial characteristics. Both ligands inhibit cell proliferation (well cell counts, shaded region). BMP2 induces a larger number of cells in clusters compared to TGFβ1 (cells per cluster, shaded region,pvalue = 0.0175). TGFβ1 causes cells to spread and have a longer distance to their second nearest neighbors (distance to second neighbors, shaded region,pvalue = 9.4032E-06). Cells grown in non-collagen-coated regular tissue-culture plates show phenotype reversal of cells per cluster and distance-to-second-neighbor metrics (unshaded regions, middle and right box plots), with no significant cell number differences between BMP2 and TGFβ1. The box edges correspond to the 25th−75th percentiles, the horizontal black lines represent the median, and the dots are individual data points. The whiskers extend to the non-outlier extremes. ns: not significant, asterisk:pvalue <0.05, three asterisks:pvalue <0.001. Significance using two-sided Student’st-test with unequal variance. Data shown are fromN= 6, 6, 8, and 4 biological replicates respectively. Source data are provided as Source Data file.eThe schematic of TGFβ1 specific regulation of a non-SMAD pathway, inferred by the MOBILE pipeline. TGFβ1 induces laminin pathway gene expression and leads to cell scattering and cell spreading with larger cells, when compared to BMP2 stimulation. 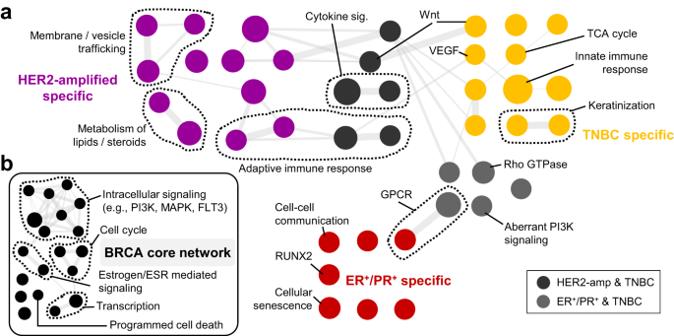Fig. 7: MOBILE infers breast cancer subtype-specific and differentially activated pathways. aThe LOGO-IANs are pair-wise compared and subtype-specific pathway enrichments are determined. The colors represent subtypes (purple: HER2-amplified, gold: TNBC, red: ER/PR-positive, gray: subtype shared), node size depends on pathway gene-set size, and edge width correlates with shared gene-set similarity of the connected nodes. Examples of pathways are labeled individually or as groups.bThe pathways enriched in all LOGO-IAN conditions constitute the breast cancer (BRCA) core network. The list includes cell cycle, estrogen, MAPK, and PI3K signaling as well as transcriptional regulation and programmed cell death. Node size and edge width represent the gene-set size and gene-set similarity of the connected nodes, respectively. The experiments were not randomized.